Single neurons in monkey prefrontal cortex encode volitional initiation of vocalizations Broca’s area in the ventrolateral prefrontal cortex (vlPFC) has a crucial role in human volitional speech production; damage to this area causes severe impairment of speech production. Lesions in PFC of monkeys, however, have only mild effects on spontaneous vocal behaviour. Non-human primate vocalizations are thus believed to constitute affective utterances processed by a subcortical network. Here in contrast to this assumption, we show that rhesus monkeys can control their vocalizations in a goal-directed way. During single-cell recordings in the vlPFC of monkeys trained to vocalize in response to visual cues, we find call-related neurons that specifically predict the preparation of instructed vocalizations. The activity of many call-related neurons before vocal output correlates with call parameters of instructed vocalizations. These findings suggest a cardinal role of the monkey homologue of Broca’s area in vocal planning and call initiation, a putative phylogenetic precursor in non-human primates for speech control in linguistic humans. Speech is one of the key distinguishing features that defines us as human, allowing us complex audio-vocal communication [1] , [2] . Learned vocal patterns such as human speech are produced primarily by cortical areas, with Broca’s area in the ventrolateral prefrontal cortex (vlPFC), comprising Brodmann areas (BA) 44 and 45 as a key structure that allows humans to voluntarily produce sophisticated speech signals. Brain damage in this region causes dysfunctions or severe impairment of speech and language production, known as Broca’s aphasia [3] , [4] . In contrast to human speech, evidence suggest that vocalizations of non-human primates may be genetically pre-programmed and generated by a complex neuronal network in the brainstem [5] , [6] , [7] . Lesions in the cortical brain structures of monkeys have no or only mild effects on spontaneous call behaviour [5] , [8] , [9] , [10] , [11] . This and other observations led to the assumption that vocalizations of non-human primates might be exclusively affective utterances bonded to specific motivational states [5] , [12] , [13] , [14] . Whether non-human primates can decouple their vocalizations from the accompanied motivational state and instrumentalize them in a goal-directed way remained a matter of debate for decades [15] , [16] , [17] . Recently, the debate was fuelled by two studies claiming to show evidence for volitional control of vocalizations in macaques and a gibbon, respectively [18] , [19] . Both studies show that monkeys are able to vocalize in response to a food reward. Thus, rather than demonstrating the capability to volitionally vocalize on command, both studies confirm that non-human primates produce adequate motivationally based responses to hedonistic stimuli. Cognitive control of non-human primate vocalizations, however, would be required to demonstrate that monkeys can be trained to reliably vocalize in response to arbitrary (that is, non-hedonic and non-social) cues in a controlled experimental protocol. In a recent study, we demonstrated that monkeys can be trained to reliably call in response to arbitrary visual stimuli [20] . Macaques thus show the minimum requirement for volitional instrumentalization of their vocalizations. Now, where in the brain could the cognitive control of calls be presented? Until now, it is largely unknown how cortical structures are involved in vocal production processes. A few studies indicate that the anterior cingulate cortex (ACC) might have a crucial role in vocal production of New and Old World monkeys [5] , [21] , [22] , [23] . Further, a recent study reported single-unit activity in the premotor cortex of macaque monkeys that preceded vocal onsets and, therefore, indicates a possible role of the premotor cortex in voluntary call initiation [18] . However, it is yet unknown how the PFC at the apex of the cortical hierarchy is involved in cognitive control of call initiation. Recent studies suggest a monkey homologue of Broca’s area (BA 44 and 45) in the vlPFC of rhesus monkeys. Although much less developed, BA 44 and 45 in macaques share a similar anatomy in terms of cytoarchitectonics and cortico-cortical connections with human Broca’s area [24] , [25] , [26] , [27] . In addition, functional commonalities have emerged over the past years. Electrical microstimulation in BA 44 elicited orofacial responses [25] , and auditory stimulation evoked distinct patterns of brain activity in BA 44 and 45 only with species-specific vocalizations in awake behaving rhesus monkeys [28] , [29] that were comparable to responses in the human Broca’s area [30] . The vlPFC might thus be ideally positioned to gain cognitive control over call initiation. In the current study, we record from BA 44 and 45 of the vlPFC in vocalizing monkeys that were trained to reliably call in response to arbitrary visual stimuli. We find vocalization-related neurons that specifically predict the preparation of instructed vocalizations in the vlPFC. The activity of many call-related neurons before the vocal output correlates with call parameters of instructed vocalizations. The comparison of neuronal responses during conditioned and spontaneous vocalizations suggests a specific involvement of the monkey homologue of Broca’s area during volitional monkey vocalizations. Volitional control on vocal onset in response to visual cues We trained two rhesus monkeys ( Macaca mulatta ) in a computer-controlled ‘go’/’nogo’ detection task to vocalize in response to the presentation of arbitrary visual stimuli (red or blue squares) to receive a reward (see Fig. 1a for experimental design). To demonstrate that the affective state associated with a call type did not influence the cognitive control of vocalizations, each monkey was trained to utter a different call type (see Fig. 1b ). One monkey (monkey T) was trained to utter ‘coo’ vocalizations (harmonic vocalization [31] ), the second monkey (monkey C) was taught to emit ‘grunts’ (noisy call [31] ). 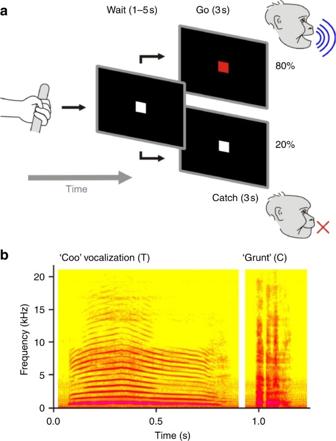Figure 1: Protocol of the go/no-go vocalization task. (a) Monkeys were trained in a go/nogo protocol to vocalize whenever a visual cue appeared. (b) Spectrograms of representative ‘coo’ and ‘grunt’ vocalizations. Monkey T uttered ‘coo’ vocalizations, whereas monkey C elicited ‘grunts’ in response to the visual cues. Spectral intensity is represented by different shades of colour. Figure 1: Protocol of the go/no-go vocalization task. ( a ) Monkeys were trained in a go/nogo protocol to vocalize whenever a visual cue appeared. ( b ) Spectrograms of representative ‘coo’ and ‘grunt’ vocalizations. Monkey T uttered ‘coo’ vocalizations, whereas monkey C elicited ‘grunts’ in response to the visual cues. Spectral intensity is represented by different shades of colour. Full size image Data from 33 daily sessions for monkey T and 27 sessions for monkey C were collected. Each session consisted of 133±8 (monkey T) and 134±6 (monkey C) vocalizations per session on average. The monkeys’ call pattern in this task was analysed with measures from the signal detection theory. In both monkeys, d ′-values were above the detection threshold in all sessions (mean d ′: 3.3±0.1 in monkey T; 4.7±0.1 in monkey C, Fig. 2a ) and show that the monkey produced calls very reliably and almost exclusively in response to the visual go-cues. Both monkeys showed similar response patterns with median call latencies of 1.50 s (monkey T) and 1.79 s (monkey C; Fig. 2b ). 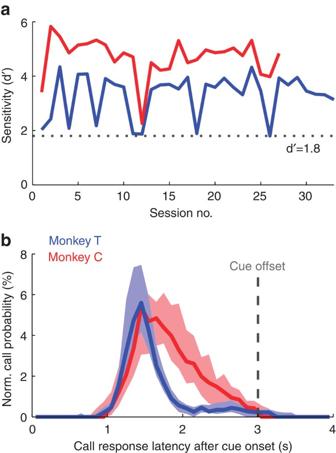Figure 2: Behavioural performance in the go/no-go vocalization task. (a) Sensitivity of vocal detection for both monkeys indexed by thed′-value (33 sessions for monkey T and 27 sessions for monkey C). The dotted line indicated the border for successful signal detection (b) Call probability of both monkeys during ‘go’ trials (normalized for 33 (monkey T) and 27 sessions (monkey C); bin width 100 ms, shaded areas indicate 1st and 3rd quartiles). Figure 2: Behavioural performance in the go/no-go vocalization task. ( a ) Sensitivity of vocal detection for both monkeys indexed by the d ′-value (33 sessions for monkey T and 27 sessions for monkey C). The dotted line indicated the border for successful signal detection ( b ) Call probability of both monkeys during ‘go’ trials (normalized for 33 (monkey T) and 27 sessions (monkey C); bin width 100 ms, shaded areas indicate 1st and 3rd quartiles). Full size image Vocalization-related neuronal activity in the frontal lobe While the monkeys performed this task, we recorded from 956 single neurons in the ventral PFC (BA 44 and 45) and the adjacent rostroventral part of the lateral premotor cortex (BA 6) to investigate whether and how these areas control the initiation of volitional vocal behaviour (see Fig. 3a,b ). To prevent putative contamination of vocalization-related activity with eye movement and/or fixation-related signals (the monkeys were not required to maintain fixation during the task), we excluded the 11.3% of neurons (108/956) that showed significant eye movement-related activity (see Fig. 4a for example neuron, Fig. 4b for neuron positions and Fig. 4c for definition) and additionally the 3.5% of neurons (33/956) that showed significant fixation-related activity (see Fig. 4d for example neuron) from all further analyses. 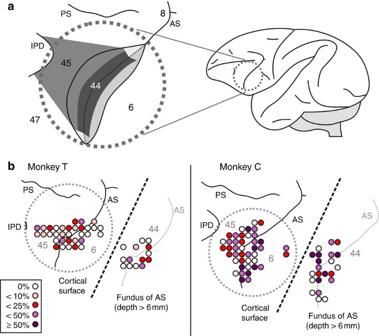Figure 3: Recording sites in vlPFC and adjacent premotor cortex of both monkeys. (a) Lateral view of the left hemisphere indicating the recording area encompassing BA 44/45 (monkey homologue of the Broca area) and adjacent BA 6 as shown in the enlarged section. (b) Precise recording sites inside each recording chamber (grey dotted circles). Recording sites with a depth >6 mm were defined as area 44 sites. For better overview, recording sites within the fundus of the inferior AS (area 44) are depicted offset on the right side of each chamber (see Methods). The proportion of the vocalization-correlated units in relation to all neurons recorded at a specific recording site is colour coded. AS, arcuate sulcus; IPD, inferior precentral dimple; PS, principal sulcus. Figure 3: Recording sites in vlPFC and adjacent premotor cortex of both monkeys. ( a ) Lateral view of the left hemisphere indicating the recording area encompassing BA 44/45 (monkey homologue of the Broca area) and adjacent BA 6 as shown in the enlarged section. ( b ) Precise recording sites inside each recording chamber (grey dotted circles). Recording sites with a depth >6 mm were defined as area 44 sites. For better overview, recording sites within the fundus of the inferior AS (area 44) are depicted offset on the right side of each chamber (see Methods). The proportion of the vocalization-correlated units in relation to all neurons recorded at a specific recording site is colour coded. AS, arcuate sulcus; IPD, inferior precentral dimple; PS, principal sulcus. 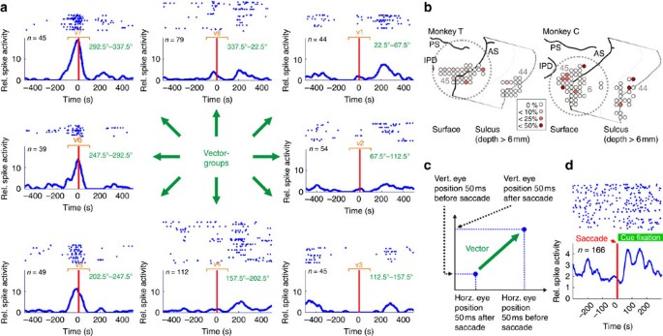Figure 4: Eye movement and fixation-correlated activity. (a) Example neuron showing direction selectivity in correlation to saccadic eye movements. Eye movement-correlated activity was calculated within a 200-ms window (v1–v8) starting 100 ms before the saccade onset throughout all eight vector groups (the Kruskal–Wallis test,P<0.05). (b) Precise recording sites inside each recording chamber (grey dotted circles) and proportion of eye movement-correlated units for both monkeys. Recording sites with a depth >6 mm were defined as area 44 sites (see Methods). The proportion of eye movement-correlated units is colour coded. AS, arcuate sulcus; IPD, inferior precentral dimple; PS, principal sulcus. (c) Saccade direction was defined as the vector of the eye position 50 ms before and 50 ms after a single saccade (c) and grouped into one of eight vector groups (seea). (d) Eye fixation-related activity. Example neuron showing significant increase in the FR during a fixation period of at least 200 ms (green bar). Eye fixation-correlated activity was calculated by comparing FRs between a 100-ms window starting 100 ms after the fixation onset and a 100-ms window just before eye fixation (the Wilcoxon-signed rank test,P<0.05). Full size image Figure 4: Eye movement and fixation-correlated activity. ( a ) Example neuron showing direction selectivity in correlation to saccadic eye movements. Eye movement-correlated activity was calculated within a 200-ms window (v1–v8) starting 100 ms before the saccade onset throughout all eight vector groups (the Kruskal–Wallis test, P <0.05). ( b ) Precise recording sites inside each recording chamber (grey dotted circles) and proportion of eye movement-correlated units for both monkeys. Recording sites with a depth >6 mm were defined as area 44 sites (see Methods). The proportion of eye movement-correlated units is colour coded. AS, arcuate sulcus; IPD, inferior precentral dimple; PS, principal sulcus. ( c ) Saccade direction was defined as the vector of the eye position 50 ms before and 50 ms after a single saccade ( c ) and grouped into one of eight vector groups (see a ). ( d ) Eye fixation-related activity. Example neuron showing significant increase in the FR during a fixation period of at least 200 ms (green bar). Eye fixation-correlated activity was calculated by comparing FRs between a 100-ms window starting 100 ms after the fixation onset and a 100-ms window just before eye fixation (the Wilcoxon-signed rank test, P <0.05). Full size image To examine neuronal response, the task phase between the go-cue onset and vocalization onset was split into an early, post-cue onset and late, pre-vocal onset analysis window. We hypothesized that neurons in the ventral prefrontal/premotor cortex that have a role in volitional initiation of vocalizations (cued vocalizations in hit trials) show different activity as compared with, first, trials in which the monkey ignored the vocalization cue (silence in miss trials) and, second, trials in which the monkey spontaneously called in the absence of a vocalization cue. We first compared the neuronal activity in cued vocalization trials (hits) with the same neurons’ responses during silent trials (misses). A proportion of 15% of recorded neurons (147/956) showed significant differences in activity (increase or decrease) during cued vocalization trials compared with silent trials in the early and/or the late analysis phase ( P <0.05, the Mann–Whitney U -test). These neurons were defined as vocalization-correlated neurons. In all three areas recorded from (BA 44, BA 45 and BA 6), monkey C showed a higher proportion of vocalization-correlated neurons (25.5%; 98/384) than monkey T (8.6%; 49/572; χ 2 -test, P <0.05). Table 1 shows the distribution of vocalization-correlated neurons recorded from each animal in each cortical area. Of those vocalization-correlated neurons, 20% (29/147) showed increased firing rates (FRs) during cued vocalization trials in the early phase ( Fig. 5a,c ) and 39% (58/147) in the late phase ( Fig. 5e,g ). Decreased discharge rates during cued vocalization trials were found in 18% (27/147) of vocalization-correlated neurons in the early ( Fig. 5b,d ) and 36% of vocalization-correlated neurons (53/147) in the late phase of cued vocalization trials ( Fig. 5f,h ). Fourteen percent of all vocalization-correlated neurons (20/147) showed differences in FRs (either increasing or decreasing) between cued vocalization and silent trials in both analysis windows. In a next step, we compared the pre-vocal activity of vocalization-correlated neurons in trials in which the monkey vocalized on command (hits) with spontaneous calls in the absence of a vocalization cue. Table 1 Numbers of vocalization-related neurons recorded from each animal in each cortical area. 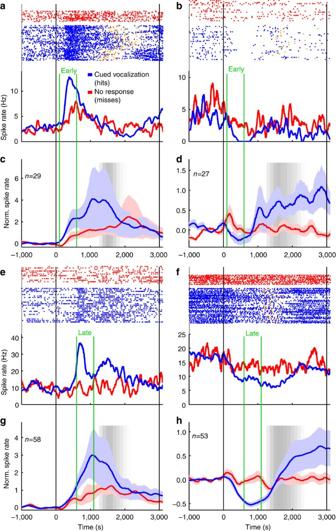Figure 5: Pre-vocal neuronal responses after cue onset. (a,b). Responses of two example neurons showing a significant increase (a; recorded in area 44) and decrease (b, area 45) of neuronal activity during trials with cued vocalizations (hits) in comparison with no response trials (misses) during the early phase right after ‘go’ onset (100–600 ms). Upper panels show raster plots, orange dots indicate vocal onset during hit trials; lower panels represent the corresponding spike density histograms averaged and smoothed with a Gaussian kernel for illustration. The vertical black lines indicate the onset and offset of the go-signal. (c,d) Averaged and normalized activity (population responses) for the corresponding examples inaandb(29 neurons forcandn=27 ford; s.e.m. is across neurons). Grey shaded areas indicate the median distributions of call onsets during hit trials. Colour shaded areas depict s.e.m. (e,f) Two example neurons showing significant increase (e, area 45) and decrease (f, area 45) of neuronal activity between hit and miss trials during the late phase just before vocal onsets. Same layout as inaandb. (g,h) Averaged and normalized activity types (population responses) for the corresponding examples ineandf. (n=58 (g) andn=53 (h); s.e.m. is across neurons). Same layout as inc. Full size table Figure 5: Pre-vocal neuronal responses after cue onset. ( a , b ). Responses of two example neurons showing a significant increase ( a ; recorded in area 44) and decrease ( b , area 45) of neuronal activity during trials with cued vocalizations (hits) in comparison with no response trials (misses) during the early phase right after ‘go’ onset (100–600 ms). Upper panels show raster plots, orange dots indicate vocal onset during hit trials; lower panels represent the corresponding spike density histograms averaged and smoothed with a Gaussian kernel for illustration. The vertical black lines indicate the onset and offset of the go-signal. ( c , d ) Averaged and normalized activity (population responses) for the corresponding examples in a and b (29 neurons for c and n =27 for d ; s.e.m. is across neurons). Grey shaded areas indicate the median distributions of call onsets during hit trials. Colour shaded areas depict s.e.m. ( e , f ) Two example neurons showing significant increase ( e , area 45) and decrease ( f , area 45) of neuronal activity between hit and miss trials during the late phase just before vocal onsets. Same layout as in a and b . ( g , h ) Averaged and normalized activity types (population responses) for the corresponding examples in e and f . ( n =58 ( g ) and n =53 ( h ); s.e.m. is across neurons). Same layout as in c . Full size image Neural differences before volitional and spontaneous calls This analysis was done in monkey T that occasionally elicited a sufficient number of spontaneous ‘coo’ vocalizations (in 17 out of 49 vocalization-correlated neurons with a mean of 11±2 spontaneous calls per neuron); monkey C never called spontaneously during recordings. First, we compared volitional ( Fig. 6a ) and spontaneous coos ( Fig. 6b ) based on their acoustical structure. We averaged spectrograms of volitional ( n =125; Fig. 6c ) and spontaneous coo vocalizations ( n =70; Fig. 6d ), which were uttered in a single daily session. Spectral analysis ( Fig. 6e ) revealed no differences between the spectrograms of volitional and spontaneous coo vocalizations for more than three-fourth of the call duration starting at vocal onset ( Fig. 6c,d ). Further, we show that the distribution of the start frequency of the calls shows no significant differences between the two call groups. Small, yet significant differences were found for call duration ( P <0.01, Wilcoxon-ranked sum test) and peak frequency ( P <0.01, Wilcoxon rank sum test), as it has been shown previously [20] (Fig. 6f ). 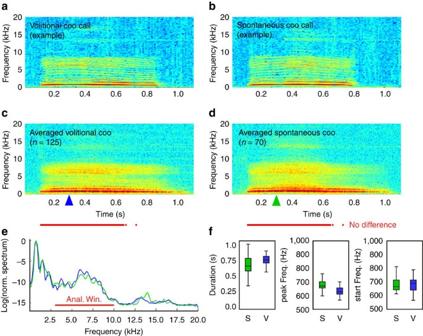Figure 6: Comparison of volitional and spontaneous coo vocalizations. (a,b) Spectrograms of two examples for a volitional and a spontaneous coo call, respectively. (c,d) Averaged spectrograms of 125 volitional and 70 spontaneous coo vocalizations uttered during a single daily session. All vocalizations are triggered on call onset. The red horizontal bar indicates the temporal region in which the averaged volitional and spontaneous coo calls show significant similarities within the analysis window (anal. win.) defined inebetween each other. (e) Examples for averaged power spectra of volitional (blue) and spontaneous vocalizations (green) calculated 0.2 s after the call onset for the spectrograms incandd, as indicated by the blue and green triangle, respectively. Colour shaded areas depict s.e.m. For statistical analysis, we focused on the frequency range between 3 and 10 kHz (anal. win.). (f) Differences in distribution of call duration, peak frequency and start frequency between volitional (V) and spontaneous (S) coo vocalizations (n=195; 125 V and 70 S calls). Medians: horizontal lines inside boxes; first and third quartiles: upper and lower margins of boxes, respectively; 5% and 95% quantile: small horizontal bars above and below boxes, respectively. Figure 6: Comparison of volitional and spontaneous coo vocalizations. ( a , b ) Spectrograms of two examples for a volitional and a spontaneous coo call, respectively. ( c , d ) Averaged spectrograms of 125 volitional and 70 spontaneous coo vocalizations uttered during a single daily session. All vocalizations are triggered on call onset. The red horizontal bar indicates the temporal region in which the averaged volitional and spontaneous coo calls show significant similarities within the analysis window (anal. win.) defined in e between each other. ( e ) Examples for averaged power spectra of volitional (blue) and spontaneous vocalizations (green) calculated 0.2 s after the call onset for the spectrograms in c and d , as indicated by the blue and green triangle, respectively. Colour shaded areas depict s.e.m. For statistical analysis, we focused on the frequency range between 3 and 10 kHz (anal. win.). ( f ) Differences in distribution of call duration, peak frequency and start frequency between volitional (V) and spontaneous (S) coo vocalizations ( n =195; 125 V and 70 S calls). Medians: horizontal lines inside boxes; first and third quartiles: upper and lower margins of boxes, respectively; 5% and 95% quantile: small horizontal bars above and below boxes, respectively. Full size image Half of the vocalization-correlated neurons during which the monkey vocalized spontaneously (47% or 8/17) showed significant differences in pre-vocal discharge rates between volitional and spontaneous vocalizations (see example neuron in Fig. 7a ). On average, vocalization-correlated neurons elicited higher pre-vocal discharge rates during volitional calls as compared with spontaneous vocalizations ( Fig. 7b ; P <0.02, the Mann–Whitney U -test, n =17). This suggests a stronger involvement of frontal areas in the initiation processes of volitional vocalizations than that of spontaneous calls. We witnessed interesting differences in the response properties of these neurons between prefrontal (BA 44/45) and premotor (BA 6) cortices ( Fig. 7c ), which was confirmed on a population level ( Fig. 7d ). First, neurons in BA 44 and 45 were characterized by high discharge rates specifically before the vocal onset, whereas BA 6 neurons showed mildly increased FRs reaching well into the vocal production phase ( Fig. 7d ). Second, maximum discharge of individual neurons was reached on average well before the vocal onset in BA 44 and BA 45 (on average 1,300 and 1,333 ms, respectively, before vocalization; Fig. 7d ), whereas neurons in BA 6 responded maximally just before the vocal onset (26 ms before vocalization; P <0.05, the Kruskal–Wallis test). These differences were due to significant differences between BA 6 and BA 44 ( P <0.05) as well as between BA 6 and BA 45 ( P <0.02); no differences were detected between BA 44 and BA 45 ( P >0.5, post hoc Mann–Whitney U -test). These results indicate that neurons in BA 44 and BA 45 are more involved in pre-vocal initiation processes, whereas BA 6 activity is more related to the actual motor output during the calling. 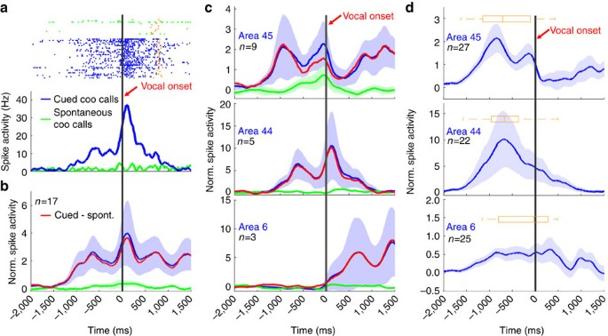Figure 7: Pre-vocal neural activity. (a) Example neuron showing significantly higher activity before vocal onset of volitional coo calls compared with spontaneous coo calls. The vertical black line indicates the onset of vocalizations. Upper panel depicts raster plots and orange dots indicate vocal offsets. Lower panel shows the corresponding spike density histograms averaged and smoothed with a Gaussian kernel for illustration. (b) Averaged and normalized neuronal activity in response to cued and spontaneous vocalizations (n=17). On average, pre-vocal discharge rates during cued vocalizations are significantly higher than during spontaneous vocalizations (P<0.02, the Mann–WhitneyU-test). Red line indicates the differences between FRs in response to cued and spontaneous calls. (c) Averaged and normalized neuronal activity of all neurons during which the monkey uttered spontaneous vocalizations (population responses) in response to cued and spontaneous vocalizations subdivided into three groups corresponding to their recording sites (area 45: 9 neurons, area 44:n=5, area 6:n=3); colour-codes as inaandb. (d) Averaged and normalized activity (population responses) of all vocalization-correlated neurons showing increased neural activity before the vocal onset (neurons showing decreased neuronal activity before the vocal onset are not shown) subdivided into three groups corresponding to their recording sites (area 45:n=27, area 44:n=22, area 6:n=25). The vertical black lines indicate the onset of vocalizations. Boxplots indicate the distribution of neural activity maxima between 2 s before and 0.5 s after the call onset of all neurons. Medians: vertical lines inside boxes; 1st and 3rd quartile: left and right margins of boxes, respectively; 5% and 95% quantile: vertical bars left and right boxes, respectively;n, number of neurons; colour shaded areas depict s.e.m. Figure 7: Pre-vocal neural activity. ( a ) Example neuron showing significantly higher activity before vocal onset of volitional coo calls compared with spontaneous coo calls. The vertical black line indicates the onset of vocalizations. Upper panel depicts raster plots and orange dots indicate vocal offsets. Lower panel shows the corresponding spike density histograms averaged and smoothed with a Gaussian kernel for illustration. ( b ) Averaged and normalized neuronal activity in response to cued and spontaneous vocalizations ( n =17). On average, pre-vocal discharge rates during cued vocalizations are significantly higher than during spontaneous vocalizations ( P <0.02, the Mann–Whitney U -test). Red line indicates the differences between FRs in response to cued and spontaneous calls. ( c ) Averaged and normalized neuronal activity of all neurons during which the monkey uttered spontaneous vocalizations (population responses) in response to cued and spontaneous vocalizations subdivided into three groups corresponding to their recording sites (area 45: 9 neurons, area 44: n =5, area 6: n =3); colour-codes as in a and b . ( d ) Averaged and normalized activity (population responses) of all vocalization-correlated neurons showing increased neural activity before the vocal onset (neurons showing decreased neuronal activity before the vocal onset are not shown) subdivided into three groups corresponding to their recording sites (area 45: n =27, area 44: n =22, area 6: n =25). The vertical black lines indicate the onset of vocalizations. Boxplots indicate the distribution of neural activity maxima between 2 s before and 0.5 s after the call onset of all neurons. Medians: vertical lines inside boxes; 1st and 3rd quartile: left and right margins of boxes, respectively; 5% and 95% quantile: vertical bars left and right boxes, respectively; n , number of neurons; colour shaded areas depict s.e.m. Full size image Call pattern-correlated neuronal activity in vlPFC Finally, we analysed whether pre-vocal activity of vocalization-correlated neurons carried information about specific call parameters. A multiple linear regression analysis was applied to test whether pre-vocal discharge rates were linked to call duration and/or peak amplitude. Sixteen percent of vocalization-correlated neurons (24/147) correlated with call patterns before the vocal onset. Out of these 24 call pattern-correlated neurons, about half (58%, or 14/24) correlated with call duration ( Fig. 8a ). Population analysis of these neurons reveal a median absolute regression slope of 5.1 ms Hz −1 ( Fig. 8c ) and a median correlation coefficient of 0.29 ( Fig. 8e ). Discharge rates of 63% of the call pattern-correlated neurons (15/24) were significantly correlated with call amplitude ( Fig. 8b ). Call amplitude-correlated neurons were characterized by a median absolute regression slope of 0.2 dB Hz −1 ( Fig. 8d ) and a median correlation coefficient of 0.24 ( Fig. 8f ) on neuronal population level. Twenty-one percent of the call pattern-correlated neurons were encoding both call duration and amplitude. Interestingly, the distribution of call pattern-correlated neurons was different between the three tested brain areas ( P <0.05, the χ 2 -test). In contrast to BA 45 with 27% of vocalization-correlated neurons encoding for call patterns, such neuronal characteristics were only found in 9% of the BA 44 cells and in 8% of BA 6 neurons ( Fig. 9a ). These results suggest a stronger involvement in vocal motor planning processes for area BA 45 than BA 44 and BA 6 ( Fig. 9b ). 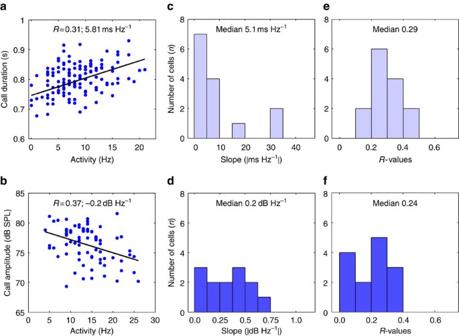Figure 8: Pre-vocal call pattern-correlated activity. (a,b) Pre-vocal FRs before vocal onset of two example neurons coding call duration (a) and call amplitude (b). Each dot depicts the neuronal activity correlated to the call pattern of a single volitional vocalization. TheR-value and negative slope are corresponding to the respective regression line. (c,d) Distribution of the absolute values of the regression slopes of neurons showing significant correlation with call duration (c) and amplitude (d). (e,f) Distribution of the correlation coefficients of neurons showing significant correlation with call duration (e) and amplitude (f). Figure 8: Pre-vocal call pattern-correlated activity. ( a , b ) Pre-vocal FRs before vocal onset of two example neurons coding call duration ( a ) and call amplitude ( b ). Each dot depicts the neuronal activity correlated to the call pattern of a single volitional vocalization. The R -value and negative slope are corresponding to the respective regression line. ( c , d ) Distribution of the absolute values of the regression slopes of neurons showing significant correlation with call duration ( c ) and amplitude ( d ). ( e , f ) Distribution of the correlation coefficients of neurons showing significant correlation with call duration ( e ) and amplitude ( f ). 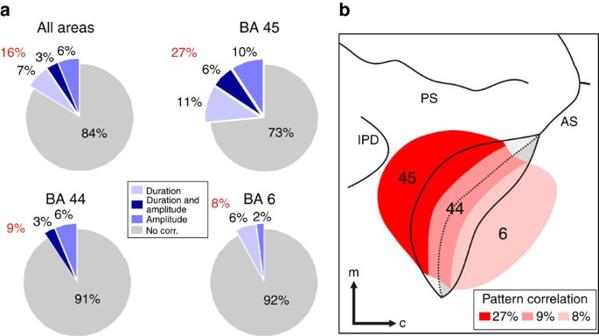Figure 9: Distribution of call pattern-correlated neurons. (a) Proportions of neurons coding duration and amplitude before vocal onset in total (n=147) and subdivided into BA44 (n=34), BA45 (n=58) and BA6 (n=55). (b) Proportion of call pattern-correlated neurons within BA45, 44 and 6 indicated by different shades of red. Full size image Figure 9: Distribution of call pattern-correlated neurons. ( a ) Proportions of neurons coding duration and amplitude before vocal onset in total ( n =147) and subdivided into BA44 ( n =34), BA45 ( n =58) and BA6 ( n =55). ( b ) Proportion of call pattern-correlated neurons within BA45, 44 and 6 indicated by different shades of red. Full size image We show that single-cell recordings in vocalizing monkeys constitute a neuronal correlate of volitional call initiation in the monkey homologue of human’s Broca area (BA 44 and 45 of the vlPFC). The activity of neurons in BA 45 before vocal onset was correlated with subsequent call duration and call amplitude. The ventral PFC might have experienced modifications during the course of primate evolution to cognitively control the subcortical vocal pattern-generating network. Our results argue for a direct involvement of BA 44/45 in motor selection and initiation processes because changes in FRs were almost exclusively present before volitional vocal onset. In addition, the fact that FRs were significantly different between volitional and spontaneous vocalizations is clear evidence that the reported discharges do not just signal orofacial components but the voluntary initiation of calls. Further, about one-fourth of neurons in BA 45 showed call pattern-correlated activity (related to call duration and call amplitude) before the vocal onset, whereas only 1 out of 12 neurons in BA 6 showed correlated activity to call patterns. Here future investigations will have to elucidate whether neurons in BA 6 show call pattern-correlated activity when call patterns are correlated with neuronal activity not long before but during the vocal output. Such pattern can be found in other brain structures that are involved in the vocal motor control such as the periaqueductal grey [32] and the ventrolateral reticular formation [6] . In contrast to cells in BA 44/45, neurons in the adjacent ventrorostral premotor cortex (BA 6vr) show peak changes in their discharge rates around the vocal onset. These findings are in agreement with the report of vocalization-correlated neurons in BA 6vr [18] and suggest a possible role of BA 6 in vocal motor-related processes rather than in vocal planning and call preparation. Differences in the fraction of neurons showing vocalization-correlated activity between both monkeys that each produced a different call type might be related to differences in cortical control for the two vocalization types. These results help to elucidate the role of frontal brain structures in the vocal motor control. Several recent studies revealed that BA 44/45 in non-human primates can be seen as a monkey’s homologue of Broca’s area [25] , which is crucial for speech control in humans [33] . BA 44/45 shows anatomical similarities, comparable cytoarchitectonics [24] as well as similar cortico-cortical projections as Broca’s area [24] . Therefore, these areas would be ideally situated to control audio-vocal behaviour [34] because they are tuned to species-specific auditory input [28] , [30] , synthesize multimodal social information [35] , [36] and generate orofacial motor output [25] . Nevertheless, a few studies report that bilateral damage to the ventrolateral frontal cortices has no significant effect on vocal behaviour in rhesus macaques [8] , [10] . However, examination of the lesion sites with recent cytoarchitectonic data [24] , [25] reveals that experimental lesions may not have included the full extent or even the bulk of BA 44/45 in these studies [8] , [10] . Moreover, lesions in vlPFC may differently affect voluntary vocalizations compared with spontaneous calls. On the basis of our results, we propose that BA 44/45 is important for vocal preparation processes, which in turn may control BA 6vr via its anatomical connections [37] , [38] , [39] . BA 6vr, directly adjacent to area 44, contains a larynx movement representation, which has been shown by electrical stimulation studies [18] , [40] , [41] , [42] . A direct control of phonatory motoneuron pools during vocal output by the larynx area of BA 6vr, however, seems to be highly unlikely. The premotor cortex in non-human primates lacks direct projections to laryngeal motoneuron pools [5] , [7] , [43] . Further, primate vocalizations are produced by an extrapyramidal neuronal network, which is coordinating the phonatory motoneuron pools by vocal pattern generators in the lower brainstem [5] , [6] . Nevertheless, the larynx area of the premotor cortex has anatomical connections to the vocal motor system on several subcortical as well as cortical levels such as the ventrolateral reticular formation, the periaqueductal grey as well as the ACC, respectively [41] , [42] , [44] . Currently, it is unknown at which processing level BA 6vr takes control over the vocal motor network during the production of volitional vocalizations. It has been suggested that a potential connection from prefrontal and premotor structures to the vocal motor network via ACC, a crucial structure during call production [5] , might be involved. Electrical stimulation elicited vocal utterances [21] , [22] and single-unit studies revealed vocalization-correlated activity that preceded the vocal onset in the ACC of macaque monkeys [23] . Further, uni- and bilateral ACC ablation only affect vocalizations uttered in an operant conditioning task, whereas the production of spontaneous calls was not disrupted [10] , [45] . These findings suggest ACC as a potential relay station between prefrontal as well as premotor structures and the vocal motor network. This previously undetected prefrontal loop for call initiation may constitute an evolutionary precursor of how networks for the generation of vocal behaviour gradually became subject to volitional control during the course of phylogeny. The prefrontal region at the apex of the cortical hierarchy processes social signals [35] and thus could be strategically situated to regulate communicative signals. Neurons in the PFC receive highly processed information to represent abstract categories [46] , [47] irrespective of sensory modality [48] . The PFC actively retrieves associative representations from long-term memory for top-down control [49] and establishes semantic associations between arbitrary items and meaningful categories [50] , [51] . However, such abstract representations and semantic associations also need to be processed according to rules and strategies to produce situational and strategic communicative utterances. Such circuitry is also hosted by the PFC because its neurons encode abstract rules [52] , [53] and sequence plans [54] , [55] . Ultimately, such neuronal circuits in the primate PFC could readily have been adopted in the course of primate evolution for processing speech and language in humans [1] , [2] . Behavioural data acquisition Stimulus presentation and behavioural monitoring was automated on personal computers running the CORTEX program (NIH) and recorded by a multiacquisition system (Plexon Inc., Dallas, TX). Vocalizations were recorded synchronously with the neuronal data by the same system with a sampling rate of 40,000 Hz via an analog-to-digital converter for post hoc analysis. A custom-written MATLAB program running on another personal computer monitored the vocal behaviour in real-time and detected vocalizations automatically by calculating online several acoustic parameters such as duration, peak frequency, amplitude, wiener entropy, chaotic index and several spectral analyses (see Table 2 for further details). By setting specific ranges for each call parameter for each call type, we were able to detect vocalizations and distinguish them from other sounds. The mean detection rate for coo vocalizations was well above 99%. Misses of coo calls did not occur. False positives were very rare with a total of 9 cases over all 33 sessions with ~4,400 calls in total. The noisy character and short duration of grunt calls made them more difficult to distinguish automatically from external ambient sounds. False positives were also rare for grunts, whereas misses of grunt vocalizations occurred occasionally and were flagged and rewarded manually online. To erase false positives, we double-checked every single trial offline audio-visually to ensure proper detection. Table 2 Ranges of acoustic parameters that were used for automatic vocal detection. Full size table Vocal on- and offset times were detected offline by a custom-written MATLAB program to assure precise timing for data analysis. Reward delivery was automatically initiated 300 ms (100 ms for grunts) after call detection, which was typically 500 ms after the call onset; thus, reward was provided no earlier than 800 ms (600 ms for grunts) after the call onset. Behavioural protocol We used two 5-year-old male rhesus monkeys ( M. mulatta ) weighing 4.2 and 4.5 kg for this study. A trial began when the monkey initiated a ‘ready’ response by grasping a bar (see Fig. 1a ). A visual cue, indicating the ‘nogo’ signal (‘pre-cue’; white square, diameter: 0.5° of visual angle) appeared for a randomized time of 1–5 s; vocal output had to be withheld during this period. Next, a coloured visual ‘go’ signal appeared in 80% of the trials (red or blue square with equal probability ( P =0.5); diameter: 0.5° of visual angle) lasting for 3,000 ms. During presentation of the ‘go’ signal, the monkey had to emit a vocalization to receive a reward (drops of water). According to the signal detection theory [56] , successful calls during ‘go’ trials were defined as ‘hits’ and vocalizations during ‘catch’ trials as ‘false alarms’. Cue colour had no influence on call probability ( P >0.05 for both monkeys; the Wilcoxon-signed rank test). In the remaining 20% of the trials, no ‘go’ signal appeared and the ‘pre-cue’ remained unchanged for another 3,000 ms (‘catch’ trial). Catch trials allowed controlling for random calling behaviour because the monkey had to withhold call production during this period. ‘Catch’ trials were not rewarded. ‘False alarms’ were indicated by visual feedback (blue screen) and by trial abort. One session was recorded per individual per day. Animals were head-fixated during the experiment maintaining a constant distance of 5 cm between the animal’s head and the microphone. During the experiments, the monkeys worked under a controlled water intake protocol. All animal handling procedures were in accordance with the guidelines for animal experimentation and authorized by the Regierungspräsidium Tübingen. We computed d ′-sensitivity values derived from the signal detection theory [56] by subtracting z -scores (normal deviates) of median ‘hit’ rates from z -scores of median ‘false alarm’ rates. Detection threshold for d ′-values was set to 1.8. Neurophysiological recordings Extracellular single-unit activity was recorded with arrays of 6–14 glass-coated tungsten microelectrodes of 1 and 2 MΩ impedance (Alpha Omega, Alpharetta GA). Microelectrode arrays were inserted each recording day using a grid with 1 mm spacing. Recordings were made in the vlPFC (BA44 and 45) and the adjacent premotor cortex (BA 6vr). Neurons were randomly selected; no attempts were made to preselect neurons for vocalization-correlated neurons. The recording sites and the position of the recording chambers were localized using stereotaxic reconstructions from individual magnetic resonance images. Signal acquisition, amplification, filtering and offline spike sorting was carried out using the Plexon system. Data analysis was accomplished using MATLAB (MathWorks, Natick, MA). We analysed all well-isolated neurons with mean discharge rate >1 Hz, recorded for at least seven hit trials and three miss trials. All surgery procedures were accomplished under aseptic conditions under general anaesthesia and were in accordance with the guidelines for animal experimentation and authorized by the Regierungspräsidium. Eye movement- and fixation-correlated neurons Eye movements were monitored by a computer-controlled infrared eye tracking system (ISCAN), sampled at 1 kHz and stored with the Plexon system for offline analysis. Because of the complex behavioural design, monkeys were not additionally trained to maintain eye position. However, we made the observation that vocalizations were typically accompanied by large eye movements. Therefore, neuronal activity was analysed post hoc to exclude eye movement and eye fixation-related neurons [57] from the database. To detect saccade-related neuronal activity, we tested whether neuronal activity during the ‘pre-cue’ period was a function of saccade direction (saccades were defined as eye positions that changed for >4° of visual angle within 4 ms). The directional vectors of the saccadic eye movement were produced by comparing the eye position 50 ms before the saccade onset and 50 ms after the saccade onset ( Fig. 4c ). Directional vectors were rearranged into eight groups ( Fig. 4a ) and peri-event-time histograms were generated. We performed a non-parametric one-way analysis of variance (the Kruskal–Wallis test) to test for significant differences in FR between vector groups within 200 ms around the saccade onset. Neurons (11.3%; 108/956) that showed saccadic eye movement-correlated activity ( Fig. 4b ) were omitted from analysis on vocalization-correlated activity. To detect fixation-related neurons, we tested all neurons that did not show saccade-related neuronal activity (neurons with saccade-related activity were already excluded). ‘Fixation neurons’ are defined as neurons that increase their FRs after cue fixation [57] . We, therefore, analysed the neuronal data during recording periods in which a cue was present (‘pre-cue’, ‘go-signal’) and the animals fixated this cue stimulus. In these epochs, we analysed all fixation period of at least 200 ms in duration (note that the animals only occasionally and rapidly fixated the cue stimuli, thus preventing longer analysis windows). We performed a Wilcoxon-signed rank test ( P <0.05) to test for significant increases of FRs during the fixation period (100–200 ms after the fixation onset) compared with FRs within a 100-ms window before. Because of this analysis, 3.5% of neurons (33/956) were defined as ‘fixation neurons’ and omitted from further analysis (see Fig. 4d for example fixation neuron). Vocalization-correlated neurons We focused our analysis on pre-vocal activity in two activity periods: an early 500-ms interval starting 100 ms after the go-cue onset and a subsequent late 500-ms interval ending 1,100 ms after the go-cue onset, yet before the vocal onset. We compared FRs within the time intervals between trials with cued vocalizations (hit trials) and silent trials in which the monkey withheld vocalizations (miss trials). We performed a Mann–Whitney U -test ( P <0.05) to analyse whether neurons showed significantly increased or decreased FRs during hit trials compared with miss trials. Neurons with significant differences in FRs in at least one of the analysis windows were determined as vocalization-correlated. As monkeys were not fixating, we had to make sure that the monkeys were aware of the go-cue and that miss trials were not just a result of ‘not seeing’ the go-cue. Therefore, eye movements were observed during the first 500 ms after the go-cue onset. Trials in which the monkeys looked <100 ms on the screen were omitted from further analysis. In very few cases, monkeys vocalized with latencies <1,100 ms in response to the go-cues ( Fig. 2b ). These trials were omitted as well. Volitional and spontaneous vocalizations During the recording, monkey T sometimes produced ‘coo’ vocalizations in between trials. These trials were uttered without an external cue and therefore defined as spontaneous vocalizations. To compare pre-vocal neuronal activity between volitional ‘coo’ calls uttered during cued vocalization trials and spontaneous ‘coos’ vocalized in between cued trials, we focused the analysis on a 1,000-ms window before the vocal onset. Included in the analysis were only neurons during which the monkey produced at least three spontaneous coo calls. We performed Mann–Whitney U -tests ( P <0.05) to analyse significant differences in FRs of single neurons between volitional and spontaneous vocalizations. Spectral analysis of coo vocalization We analysed the similarity of averaged spectrograms (fast Fourier transform: 256 points; overlap 128 points) of volitional and spontaneous vocalizations by calculating the power spectra in 3.2 ms windows that were shifted in 1.6 ms steps and tested whether these spectra were significantly correlated to each other (Pearson’s correlation, P <0.05). Time windows in the spectrograms were considered as significantly similar if at least three consecutive power spectra showed significant correlations. Further, we performed Mann–Whitney U -tests ( P <0.05) to analyse significant differences of call duration, peak frequency and start frequency between volitional and spontaneous vocalizations. Assignment of neurons to different brain areas Recording sites were localized using stereotaxic reconstructions from the individuals’ magnetic resonance images. Recordings were made from the vlPFC (BA 44 and 45) and the rostroventral lateral premotor cortex (BA 6vr), with recording well and craniotomy centred around the inferior arcuate sulcus (AS). We observed a significant change in recording properties while moving the microelectrodes deep into the inferior AS at the location of BA 44, suggesting smaller and/or more densely packed neurons. These change in neural response properties were very consistent within electrode tracts and monkeys and occurred at about 6 mm below the cortical surface. For recordings deep in the inferior AS, we thus used microelectrodes with higher impedance (2 MΩ). Smaller size of neurons and the development of a rudimentary and irregular granular layer are cytoarchitectonic characteristics of BA 44 (refs 25 , 58 , 59 ). Pre-vocal peak activity To characterize differences in pre-vocal neuronal activity between brain areas, peak activities of neurons were compared. Spike density histograms for every single neuron were averaged over trials and smoothened with a Gaussian kernel (bin width, 10 ms; step size, 1 ms). Then, the activity maximum was calculated within an analysis window starting 1,000 ms before the vocal onset and ending 500 ms after the call onset for every single neuron. Differences in the distribution of peak activities between brain areas were tested by a Kruskal–Wallis test, followed by post hoc Mann–Whitney U -tests ( P <0.05). Population analysis and normalization Normalized activity was calculated by subtracting the mean neuronal baseline activity from the neuronal responses and dividing the outcome by the s.d. of the baseline activity. For neuronal activity triggered by the go-cue onset, baseline activity was defined as the discharge rates within a time window of 100–600 ms before the corresponding go-cue onset ( Fig. 5 ). Baseline activity for neurons triggered on the call onset was defined as FRs within a time window of 100–600 ms before the corresponding go-cue onset for cued (volitional) vocalizations and a time window well outside the initiated trials for spontaneous vocalizations (1,000–1,500 ms before trial initiation; Fig. 7 ). Spike density histograms for single neurons were smoothened with a Gaussian kernel (bin width, 100 ms; step size, 1 ms) for illustrative purposes only. Multiple linear regression analysis A multiple linear regression analysis ( P <0.05) was performed to test the relationship between FR and call parameters such as duration and peak amplitude. We fitted pre-vocal neuronal activity (1,000 ms window before the vocal onset) to an arbitrary linear function of both call parameters. The FR was formulated as FR =a 0 + a dur × DUR+ a ampl × AMPL, where a dur and a ampl are the coefficients that quantify the FR dependence on duration (DUR) and peak amplitude (AMPL), respectively [60] . How to cite this article: Hage, S. R. & Nieder, A. Single neurons in monkey prefrontal cortex encode volitional initiation of vocalizations. Nat. Commun. 4:2409 doi: 10.1038/ncomms3409 (2013).